Distinct Orai-coupling domains in STIM1 and STIM2 define the Orai-activating site STIM1 and STIM2 are widely expressed endoplasmic reticulum (ER) Ca 2+ sensor proteins able to translocate within the ER membrane to physically couple with and gate plasma membrane Orai Ca 2+ channels. Although they are structurally similar, we reveal critical differences in the function of the short STIM-Orai-activating regions (SOAR) of STIM1 and STIM2. We narrow these differences in Orai1 gating to a strategically exposed phenylalanine residue (Phe-394) in SOAR1, which in SOAR2 is substituted by a leucine residue. Remarkably, in full-length STIM1, replacement of Phe-394 with the dimensionally similar but polar histidine head group prevents both Orai1 binding and gating, creating an Orai1 non-agonist. Thus, this residue is critical in tuning the efficacy of Orai activation. While STIM1 is a full Orai1-agonist, leucine-replacement of this crucial residue in STIM2 endows it with partial agonist properties, which may be critical for limiting Orai1 activation stemming from its enhanced sensitivity to store-depletion. Calcium signals controlling a vast array of cellular functions are generated through the operation of channels that either release internally stored Ca 2+ or allow external Ca 2+ entry. The endoplasmic reticulum (ER) membrane-spanning STIM proteins are key mediators and coordinators of these Ca 2+ signalling events [1] . Triggered by sensing decreased Ca 2+ stored within the ER, STIM1 undergoes an intricate activation process and translocates into ER–PM junctions where it couples with and gates the highly Ca 2+ -selective family of Orai channels in the PM [1] , [2] . The entering Ca 2+ sustains Ca 2+ oscillations, maintains Ca 2+ homoeostasis, and provides crucial long-term Ca 2+ signals controlling gene expression and cellular growth [1] , [3] . Understanding the molecular basis of STIM-mediated control over Orai channel function has important clinical implications in autoimmunity, inflammation, vascular diseases and cancer [4] , [5] , [6] . Much new information on the structure and function of STIM and Orai proteins has come to light [1] , [2] , [4] , [7] . Molecular understanding of the luminal amino-terminal Ca 2+ -sensing domain of STIM1 has provided much information on the initial triggering of STIM1 as Ca 2+ stored within the ER is depleted during Ca 2+ signalling events [8] , [9] . The cytoplasmic carboxy-terminal domain that includes the Orai-interacting site has also been structurally scrutinized. A small active fragment known as the STIM-Orai-activating region (SOAR) [10] or CRAC activation domain (CAD) [11] was identified within this cytoplasmic domain of STIM1 as the minimal sequence necessary for interaction with and activation of Orai channels. Recent crystallographic analysis of SOAR from human STIM1 reveals a well-organized tetra-helical arrangement stabilized within a dimeric configuration of two SOAR peptides [12] compatible with biochemical evidence that STIM1 is a dimer in its resting state [12] , [13] , [14] , [15] . Crystallographic data has also elucidated the Orai channel architecture, analysis of Drosophila Orai revealing a hexameric arrangement of channel subunits each of which comprises four membrane-spanning helices [16] . These analyses support strong evidence [17] , [18] , [19] , [20] that the N-terminal helices of each of the six subunits, form the channel selectivity filter and line the central Orai channel pore, surrounded by the other membrane helices. The cytoplasmic ends of the N- and C-terminal Orai membrane helices extend into the cytosol and are in close proximity with each other [16] , [21] . Both the N- and C-terminal membrane helices in Orai1 are shown to be regions of interaction with STIM1 (refs 11 , 22 ), and both are clearly necessary for STIM1-induced channel activation [22] , [23] , [24] , [25] , [26] , [27] , [28] . However, the molecular site within the STIM1 molecule that interacts with Orai channels and how it induces channel gating has remained unresolved. Similar in structure and also widely expressed, the little-studied STIM2 protein differs subtly from STIM1 in its N-terminal domain, affecting luminal Ca 2+ -sensitivity [29] and self-activation [9] , [30] , [31] . Thus, small differences in residues forming the canonical Ca 2+ -sensing EF-hand domain may explain the greater sensitivity of STIM2 to changes in ER luminal Ca 2+ (refs 29 , 32 , 33 , 34 ). In addition, differences in the rates of unfolding of the luminal N-terminal domain may underlie distinct rates of activation of STIM1 and STIM2 in response to store-depletion [8] , [9] , [30] , [31] , [32] . Significantly, it was noted also that the efficacy of coupling between STIM2 and Orai1 was considerably reduced compared with that of STIM1, and that STIM2 might function as a competitive inhibitor of STIM1-mediated Ca 2+ entry [33] , [35] , [36] . We sought to determine whether the differential Orai1-coupling efficacy of STIM1 and STIM2 might be related to structural differences in their Orai-interacting domains. While the corresponding SOAR sequence in STIM2 is highly conserved, we reveal that it has a profoundly diminished interaction with and ability to gate Orai1 channels. We narrow this distinction in Orai1 activation to a small sequence in SOAR within which substitution of a single phenylalanine in STIM1 with leucine in STIM2 confers a severe decrease in Orai1 channel-gating efficacy. This amino acid is strategically positioned at the structural apex of the SOAR domain. Remarkably, modification of this single phenylalanine within the full-length STIM1 protein with the dimensionally similar but polar histidine sidechain, prevents both Orai channel binding and gating, revealing the pivotal role of this residue in both interaction with and activation of Orai. The results not only pinpoint a crucial STIM-Orai-coupling locus, but also reveal the basis of a physiologically important distinction between STIM1 and STIM2. While STIM1 is a full Orai1-agonist, leucine-replacement of this critical residue in STIM2 endows it with partial agonist properties, likely critical for limiting Orai activation stemming from the enhanced sensitivity of STIM2 to store-depletion. SOAR1 and SOAR2 are functionally distinct In addition to small differences in the luminal N-terminal Ca 2+ -sensing domains in STIM1 and STIM2 (refs 9 , 29 , 30 , 31 ), distinctions between STIM1 and STIM2 in their apparent efficacy of Orai channel-coupling [33] , [35] , [36] prompted us to functionally compare the SOAR fragments from STIM1 (SOAR1) and STIM2 (SOAR2) ( Supplementary Fig. 1 ). Despite sharing >80% amino acid identity, expressed equally in stable Orai1-CFP-expressing HEK293 cells (HEK-Orai1 cells), their coupling to Orai1 channels was remarkably different ( Fig. 1 ). In fura-2-loaded cells with replete Ca 2+ stores, constitutive Ca 2+ entry after transient (5 min) exposure to Ca 2+ -free medium was assessed by Ca 2+ readdition. Expressed YFP-SOAR1 caused robust constitutive Ca 2+ entry rapidly blocked by 50 μM 2-APB ( Fig. 1a,c) the well-described store-operated Ca 2+ entry (SOCE) modifier [37] , [38] . In contrast, YFP-SOAR2 induced only small constitutive Ca 2+ entry that was rapidly and transiently enhanced with 2-APB ( Fig. 1b,c ), despite equal expression levels ( Fig. 1d,e ). Although YFP-SOAR1 was avidly attached to Orai1 at the PM ( Fig. 1f ) consistent with earlier observations [39] , [40] , little YFP-SOAR2 was PM-associated in HEK-Orai1 cells ( Fig. 1g , left). YFP-SOAR1 remained attached even after 2-APB treatment ( Fig. 1f ) despite blocked Ca 2+ entry; in contrast, 2-APB caused a rapid association of SOAR2 with the PM ( Fig. 1g ). Förster resonance energy transfer (FRET) analysis revealed that the resting FRET level between YFP-SOAR1 and Orai1-CFP was 2.5-fold higher than that between YFP-SOAR2 and Orai1-CFP ( Fig. 1h ). Upon 2-APB addition to YFP-SOAR1-expressing cells, the FRET level increased relatively little compared with that observed for YFP-SOAR2-expressing cells ( Fig. 1i ). Indeed, the relative fractional FRET change for YFP-SOAR2 was some fivefold higher than YFP-SOAR1 ( Fig. 1j ). Thus, despite having similar sequence and predicted secondary structure ( Fig. 2 ), SOAR1 and SOAR2 differ with respect to functional coupling with the Orai1 channel. 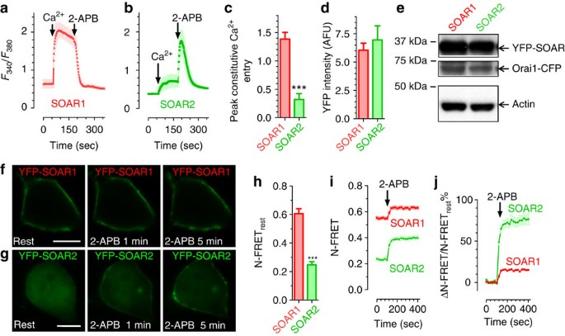Figure 1:The STIM–Orai-Activating Regions (SOAR) of STIM1 and STIM2 are functionally distinct. Fura-2 ratiometric responses to cytosolic Ca2+in HEK-Orai1 cells transiently expressing YFP-SOAR1 (a) or YFP-SOAR2 (b). SOAR-induced constitutive Ca2+entry was measured after Ca2+-free medium was replaced with 1 mM Ca2+followed by 50 μM 2-APB with 1 mM Ca2+(arrows). (c) Average peak constitutive Ca2+entry without 2-APB±s.e.m. (n≥10). (d) Average YFP fluorescence intensity (arbitrary fluorescence units; AFU) of cells in (a) and (b) ±s.e.m. (n≥10). (e) Expression of YFP-SOAR1, YFP-SOAR2 and Orai1-CFP detected with GFP antibody, compared with actin expression. (f) Cytosolic distribution of YFP-SOAR1 in HEK-Orai1 cells at rest, or 1 min or 5 min after application of 50 μM 2-APB. (g) Cellular localization of YFP-SOAR2 under the same conditions as in (f). (h–j) N-FRET between Orai1-CFP and either YFP-SOAR1 or YFP-SOAR2. (h) Mean resting N-FRET for SOAR 1 and SOAR2 (N-FRETrest) ±s.e.m. (n≥6). (i) Changes in N-FRET in response to 50 μM 2-APB. (j) N-FRET changes relative to N-FRETrestof response to 50 μM 2-APB shown in (M). Ca2+imaging and FRET responses are means±s.e.m. of multiple cells (5–17) per field. All results are typical of at least three independent experiments (***P<0.001, unpaired Student’st-test). Scale bar, 10 μm. Figure 1: The STIM–Orai-Activating Regions (SOAR) of STIM1 and STIM2 are functionally distinct . Fura-2 ratiometric responses to cytosolic Ca 2+ in HEK-Orai1 cells transiently expressing YFP-SOAR1 ( a ) or YFP-SOAR2 ( b ). SOAR-induced constitutive Ca 2+ entry was measured after Ca 2+ -free medium was replaced with 1 mM Ca 2+ followed by 50 μM 2-APB with 1 mM Ca 2+ (arrows). ( c ) Average peak constitutive Ca 2+ entry without 2-APB±s.e.m. ( n ≥10). ( d ) Average YFP fluorescence intensity (arbitrary fluorescence units; AFU) of cells in ( a ) and ( b ) ±s.e.m. ( n ≥10). ( e ) Expression of YFP-SOAR1, YFP-SOAR2 and Orai1-CFP detected with GFP antibody, compared with actin expression. ( f ) Cytosolic distribution of YFP-SOAR1 in HEK-Orai1 cells at rest, or 1 min or 5 min after application of 50 μM 2-APB. ( g ) Cellular localization of YFP-SOAR2 under the same conditions as in ( f ). ( h – j ) N-FRET between Orai1-CFP and either YFP-SOAR1 or YFP-SOAR2. ( h ) Mean resting N-FRET for SOAR 1 and SOAR2 (N-FRET rest ) ±s.e.m. ( n ≥6). ( i ) Changes in N-FRET in response to 50 μM 2-APB. ( j ) N-FRET changes relative to N-FRET rest of response to 50 μM 2-APB shown in (M). Ca 2+ imaging and FRET responses are means±s.e.m. of multiple cells (5–17) per field. All results are typical of at least three independent experiments (*** P <0.001, unpaired Student’s t -test). Scale bar, 10 μm. 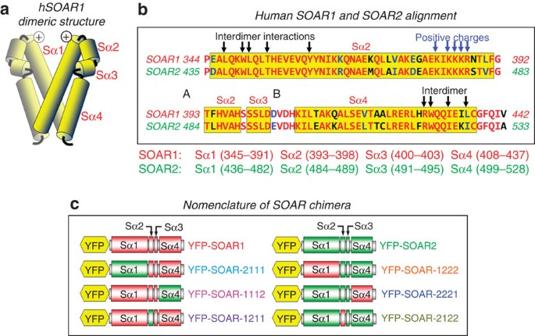Figure 2: Structure and sequence of SOAR1 and SOAR2 molecules and construction of SOAR chimeras. (a) Cartoon of dimeric human SOAR1 structure showing the four α-helices (Sα1-Sα4) as determined from the crystal structure12. (b) Alignment of human SOAR1 and SOAR2 proteins showing identical (red), conservatively differing (blue) and non-conservatively differing amino acids (black). The four α-helices are indicated by yellow boxes. Residues involved in inter-dimer interactions12are shown, as well as the positive charges that may contribute to STIM-Orai interactions25,26,53. The α-helical structure of SOAR2 is predicted to be the same as SOAR1 using homology modelling software (Biological Assembly Modeler and MolIDE; see Methods andFig. 9). (c) SOAR chimeras used in studies. The Sα1, Sα4 and Sα2 helices in SOAR1 were each individually replaced with the corresponding α-helix from SOAR2. Similarly, the Sα1, Sα4 and Sα2 helices in SOAR2 were each replaced with the corresponding α-helix from SOAR1. The chimeras generated were named according to the four α-helices they contain with α-helices from SOAR1 and SOAR2 colour coded in red and green, respectively. For example, replacement of Sα1 in SOAR1 with Sα1 from SOAR2 is named, ‘SOAR-2111’, the last four digits reflecting the origin (SOAR1 or SOAR2) or each of the four α-helices. We did not exchange Sα3 helices since they are the same; thus, the α-helices in SOAR-1122 are the same as those in SOAR-1112, and those in SOAR-2211 are the same as in SOAR-2221. The Sα2 helices differ by only one amino acid; therefore, SOAR-1211 is the same as the point mutation, SOAR1-F394L, and SOAR-2122 is the same as the point mutation, SOAR2-L485F. All chimeras were N-terminally tagged with YFP. Full size image Figure 2: Structure and sequence of SOAR1 and SOAR2 molecules and construction of SOAR chimeras. ( a ) Cartoon of dimeric human SOAR1 structure showing the four α-helices (Sα1-Sα4) as determined from the crystal structure [12] . ( b ) Alignment of human SOAR1 and SOAR2 proteins showing identical (red), conservatively differing (blue) and non-conservatively differing amino acids (black). The four α-helices are indicated by yellow boxes. Residues involved in inter-dimer interactions [12] are shown, as well as the positive charges that may contribute to STIM-Orai interactions [25] , [26] , [53] . The α-helical structure of SOAR2 is predicted to be the same as SOAR1 using homology modelling software (Biological Assembly Modeler and MolIDE; see Methods and Fig. 9 ). ( c ) SOAR chimeras used in studies. The Sα1, Sα4 and Sα2 helices in SOAR1 were each individually replaced with the corresponding α-helix from SOAR2. Similarly, the Sα1, Sα4 and Sα2 helices in SOAR2 were each replaced with the corresponding α-helix from SOAR1. The chimeras generated were named according to the four α-helices they contain with α-helices from SOAR1 and SOAR2 colour coded in red and green, respectively. For example, replacement of Sα1 in SOAR1 with Sα1 from SOAR2 is named, ‘SOAR-2111’, the last four digits reflecting the origin (SOAR1 or SOAR2) or each of the four α-helices. We did not exchange Sα3 helices since they are the same; thus, the α-helices in SOAR-1122 are the same as those in SOAR-1112, and those in SOAR-2211 are the same as in SOAR-2221. The Sα2 helices differ by only one amino acid; therefore, SOAR-1211 is the same as the point mutation, SOAR1-F394L, and SOAR-2122 is the same as the point mutation, SOAR2-L485F. All chimeras were N-terminally tagged with YFP. Full size image SOAR domains determine distinct STIM1 and STIM2 functions The stark differences between SOAR1 and SOAR2 were unexpected. We considered whether such different functions were still observed using the whole C-terminal domains from STIM1 and STIM2 in which the SOAR components operate within the larger C-terminal molecular environment ( Supplementary Fig. 1 ). Expression of the soluble cytoplasmic C-terminal domain of STIM1 (STIM1ct) reveals it to be a somewhat poor activator of Orai1 (refs 12 , 26 , 41 , 42 , 43 ). This likely results from an internal folding of the STIM1ct domain that may occlude the SOAR domain. A group of four acidic amino acids within the 318–322 sequence of STIMct (EEELE) is important in mediating this internal occlusion of STIM1ct [12] , [26] , these residues lying within a coiled-coil sequence (amino acids 310–337) described as an ‘inhibitory helix’ within STIM1ct [12] . Using HEK293 cells stably expressing CFP-Orai1 (ref. 39 ) (HEK-Orai1 cells), we expressed STIM1ct in which these four glutamates were replaced with alanines (AAALA; STIMct-4EA-YFP). Extracellular Ca 2+ add-back experiments as above revealed robust Ca 2+ entry mediated in cells expressing STIMct-4EA-YFP ( Supplementary Fig. 2a ). Addition of 50 μM 2-APB caused a brief activation followed by large inhibition of the Ca 2+ entry, consistent with its actions on STIM1-mediated SOCE in several cell types [38] . In contrast, expression of STIM2ct in which the equivalent region containing three glutamates (409–413; EQELE) were mutated to alanines (AQALA; STIM2ct-3EA-YFP) resulted in a much smaller level of constitutive Ca 2+ entry, and the addition of 50 μM 2-APB caused a rapid, large and transient activation of Ca 2+ ( Supplementary Fig. 2b ). Expression of both constructs was similar as measured by fluorescence intensity of transfected cells ( Fig. 2c ). Fluorescence imaging of the YFP-tagged proteins revealed that much STIM1ct-4EA was associated with the PM whereas there was little PM-association of STIM2ct-3EA ( Fig. 2d,e ). Considering that the large C-terminal variable regions within the STIM1ct and STIM2ct ( Supplementary Fig. 1 ) might contribute to differences in function, we deleted the entire variable regions from STIM1ct and STIM2ct and expressed the shortened STIM1ctΔV-4EA-YFP (234–505) and STIM2ctΔV-3EA-YFP (325–595) constructs. Despite elimination of these variable regions, the distinct activation of Orai channels by the two C-terminal constructs was almost exactly the same ( Fig. 3a,b ). STIM1ctΔV-4EA-YFP expression resulted in robust constitutive activation blocked by 2-APB, whereas identical expression ( Fig. 3c,d ) of STIM2ctΔV-3EA-YFP gave virtually no constitutive Ca 2+ entry but was rapidly activated by 2-APB. As with the larger whole C-terminal fragments, the STIM1ctΔV-4EA-YFP molecule was clearly visible at the plasma membrane while the STIM2ctΔV-3EA-YFP was largely cytosolic ( Fig. 3e,f ). FRET analysis of the interaction with Orai revealed that the STIM2ctΔV-3EA-YFP had a much lower basal FRET value than the STIM1ctΔV-4EA-YFP molecule ( Fig. 3g ). Upon addition of 2-APB, the STIM1-Orai1 FRET value increased by more than twofold for STIM2ctΔV-3EA-YFP whereas the value for the STIM1 construct changed by only ~20% with 2-APB ( Fig. 3h ). Clearly, the STIM2ct construct was again much poorer at interacting with and activating Orai1. These results reveal that intrinsic differences in the SOAR domains, mediate distinct functions of the entire C-terminal domains of the two STIM proteins. 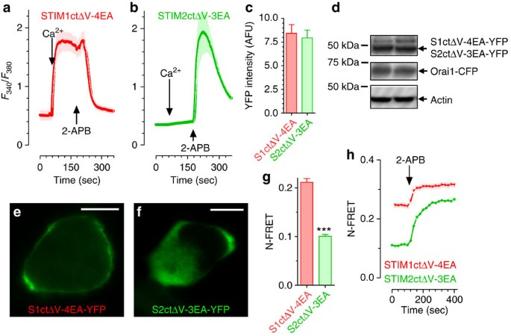Figure 3: Removal of the C-terminal variable regions from the STIM1ct and STIM2ct EA-mutants does not alter their distinct Orai1 activation and Orai1 binding properties. The STIM1 and STIM2 C-terminal constructs used inSupplementary Fig. 2were each truncated to remove their C-terminal variable regions to give the STIM1ctΔV-4EA-YFP and STIM2ctΔV-3EA-YFP, as shown inSupplementary Fig. 1. Expressed in HEK-Orai1 cells, the Ca2+responses for STIM1ctΔV-4EA-YFP (a) or STIM2ctΔV-3EA-YFP (b) are shown after 1 mM Ca2+or 50 μM 2-APB addition. Cells expressed almost equal levels of YFP fluorescence (c; means±s.e.m.), and Western analysis revealed similar protein levels (d) detected with GFP antibody. Cytosolic distribution of STIM1ctΔV-4EA-YFP (e) or STIM2ctΔV-3EA-YFP (f) at rest. (g) Resting N-FRET levels between Orai1-CFP and STIM1ctΔV-4EA-YFP (red) or STIM2ctΔV-3EA-YFP (green) (P<0.001 (n≥6) and changes in N-FRET following 50 μM 2-APB application (h). Ca2+imaging and FRET responses are means±s.e.m. of multiple cells (7–26) per field. Results are typical of at least three independent experiments (***P<0.001, unpaired Student’st-test). Scale bar, 10 μm. Figure 3: Removal of the C-terminal variable regions from the STIM1ct and STIM2ct EA-mutants does not alter their distinct Orai1 activation and Orai1 binding properties. The STIM1 and STIM2 C-terminal constructs used in Supplementary Fig. 2 were each truncated to remove their C-terminal variable regions to give the STIM1ctΔV-4EA-YFP and STIM2ctΔV-3EA-YFP, as shown in Supplementary Fig. 1 . Expressed in HEK-Orai1 cells, the Ca 2+ responses for STIM1ctΔV-4EA-YFP ( a ) or STIM2ctΔV-3EA-YFP ( b ) are shown after 1 mM Ca 2+ or 50 μM 2-APB addition. Cells expressed almost equal levels of YFP fluorescence ( c ; means±s.e.m. ), and Western analysis revealed similar protein levels ( d ) detected with GFP antibody. Cytosolic distribution of STIM1ctΔV-4EA-YFP ( e ) or STIM2ctΔV-3EA-YFP ( f ) at rest. ( g ) Resting N-FRET levels between Orai1-CFP and STIM1ctΔV-4EA-YFP (red) or STIM2ctΔV-3EA-YFP (green) ( P <0.001 ( n ≥6) and changes in N-FRET following 50 μM 2-APB application ( h ). Ca 2+ imaging and FRET responses are means±s.e.m. of multiple cells (7–26) per field. Results are typical of at least three independent experiments (*** P <0.001, unpaired Student’s t -test). Scale bar, 10 μm. Full size image SOAR1/SOAR2 chimeras reveal the crucial Orai-activating site The distinct functions of the SOAR domains not only revealed fundamental differences in Orai coupling between STIM1 and STIM2, they also provided a valuable strategy to identify the molecular site on STIM proteins mediating Orai channel activation. The recent human SOAR1 crystal structure reveals a dimeric configuration [12] compatible with biochemical evidence that resting STIM1 is a dimer [12] , [15] . Each SOAR1 monomer comprises a group of four α-helices [12] . We constructed SOAR1/SOAR2 chimera in which we exchanged each of these α-helical sequences (Sα1-Sα4) ( Fig. 2 ). Compared with wild-type-SOAR1 and SOAR2 ( Fig. 4a,b ), a chimera in which the Sα1 helix in SOAR1 was replaced with Sα1 from SOAR2 (SOAR-2111; Fig. 4c ), behaved like SOAR2 giving low constitutive Ca 2+ entry that was activated by 2-APB. Its largely cytoplasmic location and low basal FRET activated by 2-APB were also similar to SOAR2. The reciprocal chimera, SOAR-1222 in which Sα1 from SOAR1 was substituted within SOAR2, took on an interesting mixed phenotype ( Fig. 4d ). Like SOAR2, the constitutive Ca 2+ entry mediated by SOAR-1222 was low and sharply activated by 2-APB. However, unlike SOAR2, SOAR-1222 was tightly PM-associated and FRET between Orai1-CFP and YFP-SOAR-1222 was high and changed little with 2-APB, resembling SOAR1. The constitutive Ca 2+ entry (summary in Fig. 4g ), resting FRET (summary in Fig. 4h ), and cytosolic distribution, indicate that the Sα1 helix confers SOAR1 with the ability to strongly bind Orai1, whereas at least part or all of the remaining α-helices from SOAR1 contribute to its greater efficacy of channel activation. 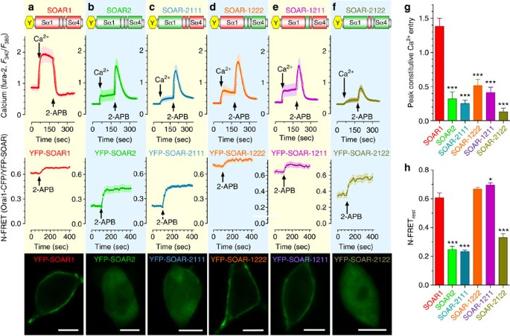Figure 4:The Sα1 and Sα2 helices of SOAR1 and SOAR2 crucially determine differences in binding and activation of the Orai1 channel. Comparative function of YFP-SOAR1 (a), YFP-SOAR2 (b), the Sα1-exchanged chimeras, YFP-SOAR-2111 (c) and YFP-SOAR-1222 (d), and the Sα2-exchanged chimeras, YFP-SOAR-1211 (e) and YFP-SOAR-2122 (f), expressed in HEK-Orai1 cells. Fura-2 measurements (upper row) were in Ca2+-free medium with addition of 1 mM extracellular Ca2+and 50 μM 2-APB (arrows). FRET measurements (middle row) were with 1 mM Ca2+with 50 μM 2-APB added (arrows). Deconvolved images of YFP-SOAR distribution (lower row) were with 1 mM Ca2+. (g) Mean of peak Ca2+entry without 2-APB±s.e.m. (n≥6). (h) Mean of resting N-FRET±s.e.m. (n≥5). *** differences from SOAR1,P<0.001 (unpaired Student’st-test). Ca2+imaging and FRET results are means±s.e.m. of multiple cells (5–17) per field, typical of at least three independent experiments. Scale bar, 10 μm. Figure 4: The S α 1 and S α 2 helices of SOAR1 and SOAR2 crucially determine differences in binding and activation of the Orai1 channel. Comparative function of YFP-SOAR1 ( a ), YFP-SOAR2 ( b ), the Sα1-exchanged chimeras, YFP-SOAR-2111 ( c ) and YFP-SOAR-1222 ( d ), and the Sα2-exchanged chimeras, YFP-SOAR-1211 ( e ) and YFP-SOAR-2122 ( f ), expressed in HEK-Orai1 cells. Fura-2 measurements (upper row) were in Ca 2+ -free medium with addition of 1 mM extracellular Ca 2+ and 50 μM 2-APB (arrows). FRET measurements (middle row) were with 1 mM Ca 2+ with 50 μM 2-APB added (arrows). Deconvolved images of YFP-SOAR distribution (lower row) were with 1 mM Ca 2+ . ( g ) Mean of peak Ca 2+ entry without 2-APB±s.e.m. ( n ≥6). ( h ) Mean of resting N-FRET±s.e.m. ( n ≥5). *** differences from SOAR1, P <0.001 (unpaired Student’s t -test). Ca 2+ imaging and FRET results are means±s.e.m. of multiple cells (5–17) per field, typical of at least three independent experiments. Scale bar, 10 μm. Full size image We next considered the role of the two small intervening α-helices, Sα2 and Sα3, within SOAR. The 4-amino-acid Sα3 helix is identical within SOAR1 and SOAR2. However, the 6-amino-acid Sα2 helix has one amino-acid difference; phenylalanine (F394) in SOAR1 is a leucine residue in SOAR2 (L485). Hence, we constructed the YFP-SOAR-1211 chimera simply by making the F394L point mutation in SOAR1. This single substitution in SOAR1 led to a profoundly different phenotype when expressed in HEK-Orai1 cells. Compared with SOAR1, the SOAR-1211 chimera ( Fig. 4e,g ) induced much lower constitutive Ca 2+ entry that was enhanced with 2-APB, much like SOAR2. Yet, SOAR-1211 was mostly PM-associated and FRET between YFP-SOAR-1211 and Orai1-CFP was high and barely altered by 2-APB ( Fig. 4e,h ), similar to that for SOAR1. In the reciprocal experiment, we made the L485F point mutation in SOAR2 to create the SOAR-2122 chimera. Although its expression was lower than SOAR2, its phenotype appeared similar to SOAR2 with respect to low constitutive Ca 2+ entry activated by 2-APB, mostly cytoplasmic expression, and relatively low FRET enhanced by 2-APB ( Fig. 4f–h ). Thus, the diminished Orai1 binding conferred on SOAR-2122 by virtue of its STIM2 Sα1 helix, was dominant in preventing its activation of Orai1. We also substituted the Sα4 helices between SOAR1 and SOAR2 and expressed these chimeras in stable HEK-Orai1 cells. However, the Sα4 substitutions (SOAR-1112 and SOAR-2221) did not change SOAR1 or SOAR2 function ( Fig. 5 ). Thus, like SOAR1, SOAR-1112 expression led to large Ca 2+ entry that was blocked by 2-APB ( Fig. 5a,c,e,f ). Also like SOAR1, SOAR-1112 was PM-associated, and FRET between SOAR-1112 and Orai1-CFP was high and relatively unchanged by 2-APB. Conversely, SOAR-2221 behaved in Ca 2+ imaging, cytoplasmic distribution, and FRET, much like SOAR2 ( Fig. 5b–f ). Thus, the Sα4 helices in SOAR1 and SOAR2 function similarly and do not contribute to the distinct characteristics of these proteins. 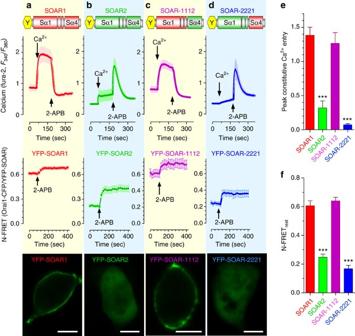Figure 5: The Sα4 helices of SOAR1 and SOAR2 do not contribute to their distinct binding properties or activation of the Orai1 channel. Comparative function of YFP-SOAR1 (a), YFP-SOAR2 (b) and the Sα4-exchanged chimeras, YFP-SOAR-1112 (c) and YFP-SOAR-2221 (d), expressed in HEK-Orai1 cells. Fura-2 measurements (upper row) were in Ca2+-free medium with addition of 1 mM extracellular Ca2+and 50 μM 2-APB (arrows). FRET measurements (middle row) were with 1 mM Ca2+with 50 μM 2-APB added (arrows). Deconvolved images of YFP-SOAR distribution (lower row) were with 1 mM Ca2+. (e) Mean of peak Ca2+entry without 2-APB ±s.e.m. (n≥7). (f) Mean of resting N-FRET ±s.e.m. (n≥4). *** differences from SOAR1,P<0.001, unpaired Student’st-test. Ca2+imaging and FRET responses are means±s.e.m. of multiple cells (5–20) per field and all results are typical of at least 3 independent experiments. Scale bar, 10 μm. Figure 5: The Sα4 helices of SOAR1 and SOAR2 do not contribute to their distinct binding properties or activation of the Orai1 channel. Comparative function of YFP-SOAR1 ( a ), YFP-SOAR2 ( b ) and the Sα4-exchanged chimeras, YFP-SOAR-1112 ( c ) and YFP-SOAR-2221 ( d ), expressed in HEK-Orai1 cells. Fura-2 measurements (upper row) were in Ca 2+ -free medium with addition of 1 mM extracellular Ca 2+ and 50 μM 2-APB (arrows). FRET measurements (middle row) were with 1 mM Ca 2+ with 50 μM 2-APB added (arrows). Deconvolved images of YFP-SOAR distribution (lower row) were with 1 mM Ca 2+ . ( e ) Mean of peak Ca 2+ entry without 2-APB ±s.e.m. ( n ≥7). ( f ) Mean of resting N-FRET ±s.e.m. (n≥4). *** differences from SOAR1, P <0.001, unpaired Student’s t -test. Ca 2+ imaging and FRET responses are means±s.e.m. of multiple cells (5–20) per field and all results are typical of at least 3 independent experiments. Scale bar, 10 μm. Full size image STIM activation of Orai is tuned by a single amino acid The results from the Sα2 chimera reveal that the single phenylalanine-394 residue in the Sα2 helix of SOAR1 is a crucial locus for the induction of Orai1 channel opening. Considering SOAR exposure and function within STIM1 is a complex and highly controlled process [1] , we asked whether the F394 residue plays a similar role in the full-length STIM protein environment. Certainly, SOAR1 and SOAR2 function is preserved within their expressed whole C-terminal domains ( Fig. 3 , Supplementary Fig. 2 ). Important was to examine the role of F394 within the intact STIM1 protein. Compared with STIM1-wt, equal expression of the F394L mutation in HEK-Orai1 cells resulted in substantially reduced SOCE ( Figs 6a,b and 7a ). Diminishing the side-chain size of the hydrophobic F394 residue even further to alanine (F394A), decreased the Ca 2+ entry yet further. Remarkably, mutation of the phenylalanine to histidine (F394H) to introduce polarity while preserving side-chain size, completely abolished SOCE. These STIM1 mutants did not change ionomycin-induced Ca 2+ release and hence did not alter either size or releasability of Ca 2+ stores. With all STIM1 mutants, 2-APB addition after Ca 2+ readdition rapidly induced Ca 2+ entry, indicating Orai1 channels were activatable even though store-depletion was not sufficient for activation. Using identically transfected HEK-Orai1 cells but without depleting stores, no Ca 2+ entry was observed upon Ca 2+ readdition, nor was there any 2-APB induced Ca 2+ entry ( Fig. 6c ). Thus, 2-APB overcomes the deficit in Orai1-coupling but still requires STIM1 activation by store-depletion. Patch-clamp measurements revealed that the Ca 2+ entry in response to each STIM1 mutant was mediated by authentic CRAC current ( Figs 6d–h and 7c ). 2-APB enhanced or restored CRAC current in each case ( Figs 6i and 7d ). 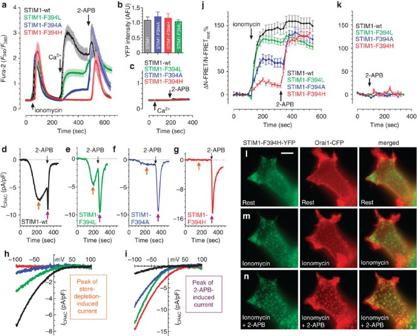Figure 6:The F394 residue within full-length STIM1 functions as a pivotal locus for both binding to and gating of Orai1 channels. (a) Fura-2 Ca2+measurements undertaken on HEK-Orai1 cells expressing wild-type STIM1-YFP (black), or STIM1 mutants F394L-YFP (green), F394A-YFP (blue), or F394H-YFP (red). Cells in Ca2+-free medium were treated with 2.5 μM ionomycin, 1 mM Ca2+and 50 μM 2-APB (arrows). (b) Average±s.e.m. YFP fluorescence intensity of cells in (a). (c) Measurements as in (a) but without ionomycin addition. (d–g) Whole-cellICRACmeasurements on HEK-Orai1 cells transfected with wild-type STIM1-YFP (d) or the STIM1 mutants, F394L-YFP (e), F394A-YFP (f) or F394H-YFP (g); currents were induced by passive store-depletion with 20 mM EGTA in the pipette, and subsequent addition of 50 μM 2-APB in the bath. Typical traces are shown of whole-cell currents at −100 mV. (h,i) I-V relationship from cells shown in (d–g) either at peak store-operated current (orange arrow) or peak 2-APB induced current (purple arrow). (j) N-FRET change between Orai1-CFP and STIM1-YFP using the same mutants expressed within HEK-Orai1 cells, as in (a). Additions of 2.5 μM ionomycin and 50 μM 2-APB in Ca2+-free medium were as shown. (k) N-FRET measurements as in (j) but without ionomycin addition. (l–n) Cytosolic distribution of Orai1-CFP (red) and STIM1-F394H-YFP (green) expressed in HEK-Orai1 cells. Images are of a single cell before (l), and after 5 min treatment with 2.5 μM ionomycin (m) and a further 5 min with 50 μM 2-APB (n). Detailed quantitative analysis and statistics on Ca2+entry, FRET, peak ICRAC and Orai1/STIM1transocation into puncta are given inFig. 7. Ca2+imaging and FRET responses are means±s.e.m. of multiple cells (8-33) per field and results are all typical of at least three independent experiments. Scale bar, 10 μm. Figure 6: The F394 residue within full-length STIM1 functions as a pivotal locus for both binding to and gating of Orai1 channels . ( a ) Fura-2 Ca 2+ measurements undertaken on HEK-Orai1 cells expressing wild-type STIM1-YFP (black), or STIM1 mutants F394L-YFP (green), F394A-YFP (blue), or F394H-YFP (red). Cells in Ca 2+ -free medium were treated with 2.5 μM ionomycin, 1 mM Ca 2+ and 50 μM 2-APB (arrows). ( b ) Average±s.e.m. YFP fluorescence intensity of cells in ( a ). ( c ) Measurements as in ( a ) but without ionomycin addition. ( d – g ) Whole-cell I CRAC measurements on HEK-Orai1 cells transfected with wild-type STIM1-YFP ( d ) or the STIM1 mutants, F394L-YFP ( e ), F394A-YFP ( f ) or F394H-YFP ( g ); currents were induced by passive store-depletion with 20 mM EGTA in the pipette, and subsequent addition of 50 μM 2-APB in the bath. Typical traces are shown of whole-cell currents at −100 mV. ( h , i ) I-V relationship from cells shown in ( d – g ) either at peak store-operated current (orange arrow) or peak 2-APB induced current (purple arrow). ( j ) N-FRET change between Orai1-CFP and STIM1-YFP using the same mutants expressed within HEK-Orai1 cells, as in ( a ). Additions of 2.5 μM ionomycin and 50 μM 2-APB in Ca 2+ -free medium were as shown. ( k ) N-FRET measurements as in ( j ) but without ionomycin addition. ( l – n ) Cytosolic distribution of Orai1-CFP (red) and STIM1-F394H-YFP (green) expressed in HEK-Orai1 cells. Images are of a single cell before ( l ), and after 5 min treatment with 2.5 μM ionomycin ( m ) and a further 5 min with 50 μM 2-APB ( n ). Detailed quantitative analysis and statistics on Ca 2+ entry, FRET, peak ICRAC and Orai1/STIM1transocation into puncta are given in Fig. 7 . Ca 2+ imaging and FRET responses are means±s.e.m. of multiple cells (8-33) per field and results are all typical of at least three independent experiments. Scale bar, 10 μm. 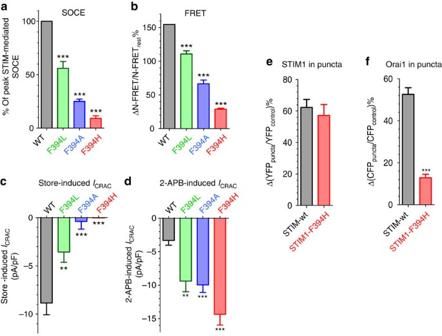Figure 7:Summary data for the effects of STIM1-F394 mutants on SOCE, Orai1 N-FRET,ICRAC, and punctal changes, shown inFig. 6. (a) Comparison of peak ionomycin-induced SOCE in HEK-Orai1 cells transfected with STIM1-YFP, STIM1-F394L-YFP, STIM1-F394A-YFP or STIM1-F394H-YFP as shown inFig. 6a(***P<0.001, unpaired Student’st-test,n=6). (b) Ionomycin-induced peak ΔN-FRET/N-FRETrest(%) with the same STIM1-YFP constructs used in (a), as shown inFig. 6j(***P<0.001, unpaired Student’st-test,n≥4). (c) PeakICRACactivity in HEK-Orai1 cells transfected with the same STIM1-YFP constructs used in (a) in response to passive store-depletion, as shown inFig. 6d–g. (d) AdditionalICRACactivity induced by 2-APB in the same cells as shown in (c) (**P<0.01; ***P<0.001; unpaired Student’st-test, WTn=6; F394Ln=4; F394An=4; F394Hn=6). (e,f) Quantitative analysis of ionomycin-induced STIM1-F394H-YFP and Orai1 movement into puncta (red; data inFig. 6l,m) compared with movement of wild-type-STIM-YFP in HEK-Orai cells (black). For STIM1 (e) the Δ(YFPpuncta/YFPcontrol)% values for wild-type STIM1-YFP and STIM1-F394H-YFP are similar. For Orai1 (f), the Δ(CFPpuncta/CFPcontrol)% for cells expressing STIM1-F394H-YFP is substantially reduced compared with cells expressing wild-type STIM1. Thus, the STIM1-F394H mutant has substantially reduced Orai-binding activity (means±s.e.m., ***P<0.001; unpaired Student’st-test). Full size image Figure 7: Summary data for the effects of STIM1-F394 mutants on SOCE, Orai1 N-FRET, I CRAC , and punctal changes, shown in Fig. 6 . ( a ) Comparison of peak ionomycin-induced SOCE in HEK-Orai1 cells transfected with STIM1-YFP, STIM1-F394L-YFP, STIM1-F394A-YFP or STIM1-F394H-YFP as shown in Fig. 6a (*** P <0.001, unpaired Student’s t- test, n =6). ( b ) Ionomycin-induced peak ΔN-FRET/N-FRET rest (%) with the same STIM1-YFP constructs used in ( a ), as shown in Fig. 6j (*** P <0.001, unpaired Student’s t -test, n ≥4). ( c ) Peak I CRAC activity in HEK-Orai1 cells transfected with the same STIM1-YFP constructs used in ( a ) in response to passive store-depletion, as shown in Fig. 6d–g . ( d ) Additional I CRAC activity induced by 2-APB in the same cells as shown in ( c ) (** P <0.01; *** P <0.001; unpaired Student’s t- test, WT n =6; F394L n =4; F394A n =4; F394H n =6). ( e , f ) Quantitative analysis of ionomycin-induced STIM1-F394H-YFP and Orai1 movement into puncta (red; data in Fig. 6l,m ) compared with movement of wild-type-STIM-YFP in HEK-Orai cells (black). For STIM1 ( e ) the Δ(YFP puncta /YFP control )% values for wild-type STIM1-YFP and STIM1-F394H-YFP are similar. For Orai1 ( f ), the Δ(CFP puncta /CFP control )% for cells expressing STIM1-F394H-YFP is substantially reduced compared with cells expressing wild-type STIM1. Thus, the STIM1-F394H mutant has substantially reduced Orai-binding activity (means±s.e.m., *** P <0.001; unpaired Student’s t -test). Full size image These results reveal the strategic significance of the STIM1-F394 residue in Orai1 channel activation. Analysis of FRET between STIM1-YFP and Orai1-CFP reveals this amino acid also has a critical role in coupling to Orai1 ( Figs 6j and 7b ). The F394L mutation had only a slight effect on store-depletion-mediated FRET between STIM1-YFP and Orai1-CFP. However, STIM1-Orai1 FRET was greatly decreased with the STIM1-F394A mutant and almost abrogated with the STIM1-F394H mutation. In both cases, 2-APB restored the STIM1-Orai1 FRET almost to the maximal levels seen with wild-type STIM1. These FRET changes were entirely dependent on store-depletion, no FRET changes occurring without ionomycin treatment, even upon 2-APB addition ( Fig. 6k ). The role of F394 in Orai1 binding was clearly observable in STIM1-YFP/Orai1-CFP localization experiments ( Fig. 6l–n ). Thus, we observed that, although the STIM1-F394H mutation still underwent store-depletion-induced puncta formation, it barely altered Orai1 distribution ( Figs 6l,m and 7e,f ). However, 2-APB restored the STIM1-Orai1 interaction and Orai1 now appeared within puncta ( Fig. 6n ). Thus, the modest F394H mutation profoundly alters the STIM1-Orai1 interaction in addition to entirely eliminating Orai1 gating. Importantly, STIM1-Orai1 antibody immunoprecipitation studies reveal the F394 residue in STIM1 critically determines the interaction between STIM1 and Orai1 ( Fig. 8 ). When expressed in normal HEK293 cells, the F394A and F394H STIM1 mutants functionally repressed endogenous SOCE ( Supplementary Fig. 4 ). Indeed, the F394H mutant in particular functioned as a powerful dominant negative. 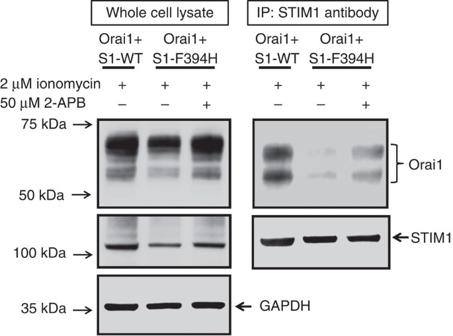Figure 8: The F394 residue critically determines binding between STIM1 and Orai1. Immunoprecipitation experiments were undertaken in HEK cells stably expressing either Orai1-CFP and STIM1-YFP (S1-WT), or Orai1-CFP and STIM1-F394H-YFP (S1-F394H). Cells were treated as indicated before lysis. Whole-cell lysates (left) and STIM1 antibody immunoprecipitates (right) are shown. Detection utilized either STIM1 antibody or GFP antibody to detect Orai1-CFP. Whereas STIM1-WT pulls down Orai1 (right, lane 1), the S1-F394H mutation is almost devoid of Orai1 interaction (right, lane 2). 2-APB enhances the interaction between S1-F394H and Orai1 after ionomycin treatment (right, lane 3). Original membrane scans are provided inSupplementary Fig. 3. Figure 8: The F394 residue critically determines binding between STIM1 and Orai1. Immunoprecipitation experiments were undertaken in HEK cells stably expressing either Orai1-CFP and STIM1-YFP (S1-WT), or Orai1-CFP and STIM1-F394H-YFP (S1-F394H). Cells were treated as indicated before lysis. Whole-cell lysates (left) and STIM1 antibody immunoprecipitates (right) are shown. Detection utilized either STIM1 antibody or GFP antibody to detect Orai1-CFP. Whereas STIM1-WT pulls down Orai1 (right, lane 1), the S1-F394H mutation is almost devoid of Orai1 interaction (right, lane 2). 2-APB enhances the interaction between S1-F394H and Orai1 after ionomycin treatment (right, lane 3). Original membrane scans are provided in Supplementary Fig. 3 . Full size image The unexpected distinction we reveal between the active sites of STIM1 and STIM2 not only has major physiological implications, but has allowed us to pinpoint the crucial Orai-coupling locus in STIM proteins. From the SOAR1 crystal structure, F394 is strategically located at the SOAR1 apex [12] with high accessibility to Orai channels ( Fig. 9a ). Homology modelling of SOAR2 predicts it has an almost identical structure to SOAR1 ( Fig. 9a,b ). SOAR1 is known to interact with both the N- and C-termini of Orai1 channels and binding across both termini is predicted to mediate channel opening [11] . SOAR1 strongly interacts with the C-terminal cytoplasmic extension of the fourth membrane-spanning helix of Orai1 (M4-extension) [11] , [12] , [22] , [23] , [24] , [25] , [26] , [28] . The positively charged region within the Sα1 helix of SOAR1 (382–387; KIKKKR; Fig. 2b ) may contribute to this strong Orai1 binding perhaps through electrostatic interactions with the Orai1 C-terminus [12] , [25] , [26] . Our SOAR chimera results reveal the Sα1 helix is critical for Orai1 binding. The STIM1-Sα1 helix confers strong Orai1 binding when inserted into SOAR2, whereas the STIM2-Sα1 helix prevents Orai1 binding when placed in SOAR1 ( Fig. 4 ). Since the positively charged residues are identical in STIM1 and STIM2 ( Fig. 2b ), the substantial difference in binding must be conferred by other amino acids. 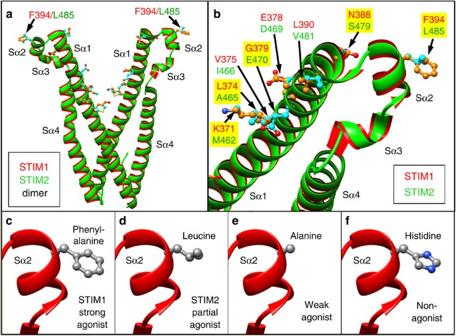Figure 9: Structural configuration of the distinct Orai-coupling domains of STIM1 and STIM2. (a) Structural comparison between SOAR1 and SOAR2 dimers. The structure of SOAR1 is derived from the crystal structure12(red). Homology modelling of residues in SOAR2 using the Biological Assembly Modeler (BAM) and MolIDE software (green) reveal the backbone ribbons for SOAR1 and SOAR2 superimpose almost exactly throughout the two molecules. The model shows only the sidechains present in the apical Sα1/Sα2 regions that differ between SOAR1 and SOAR2 (these are identified inb). SOAR1 sidechains are shown as orange, SOAR2 as light blue. (b) Detail from (a) of the two apical domains of SOAR1 and SOAR2 identifying the eight amino acids that differ in this region—seven residues in Sα1 and one in Sα2 are shown. The four non-conservative changes (K371/M462, L374/A465, G379/E470, N388/S479; yellow shaded) may contribute to the differential Orai-binding of STIM1 and STIM2. The F394/L485 substitution in Sα2 is crucial for gating differences between STIM1 and STIM2. (c–f) Structural modelling to show preferred rotamers of STIM1-F394 substituted sidechains: (c) phenylalanine (in STIM1) functions as a strong Orai agonist; (d) leucine (in STIM2) functions as a partial agonist; (e) alanine, functions as a weak agonist; (f) histidine, functions as a non-agonist. Figure 9: Structural configuration of the distinct Orai-coupling domains of STIM1 and STIM2. ( a ) Structural comparison between SOAR1 and SOAR2 dimers. The structure of SOAR1 is derived from the crystal structure [12] (red). Homology modelling of residues in SOAR2 using the Biological Assembly Modeler (BAM) and MolIDE software (green) reveal the backbone ribbons for SOAR1 and SOAR2 superimpose almost exactly throughout the two molecules. The model shows only the sidechains present in the apical Sα1/Sα2 regions that differ between SOAR1 and SOAR2 (these are identified in b ). SOAR1 sidechains are shown as orange, SOAR2 as light blue. ( b ) Detail from ( a ) of the two apical domains of SOAR1 and SOAR2 identifying the eight amino acids that differ in this region—seven residues in Sα1 and one in Sα2 are shown. The four non-conservative changes (K371/M462, L374/A465, G379/E470, N388/S479; yellow shaded) may contribute to the differential Orai-binding of STIM1 and STIM2. The F394/L485 substitution in Sα2 is crucial for gating differences between STIM1 and STIM2. ( c – f ) Structural modelling to show preferred rotamers of STIM1-F394 substituted sidechains: ( c ) phenylalanine (in STIM1) functions as a strong Orai agonist; ( d ) leucine (in STIM2) functions as a partial agonist; ( e ) alanine, functions as a weak agonist; ( f ) histidine, functions as a non-agonist. Full size image SOAR1 undergoes a second weaker interaction with the 73–85 amino-acid N-terminal segment of Orai1 (refs 11 , 22 , 23 , 24 , 44 ). This Orai1 region is a helical extension of the M1 pore-forming transmembrane helix shown by crystallography to protrude into the cytosol [16] . The interaction of SOAR with this sequence is likely key to Orai1 channel gating [11] , [21] , [22] , [23] , [24] , [27] , [28] . Our chimera experiments reveal that the Sα2 helix is crucial for Orai1 channel gating ( Fig. 4 ). Substitution of STIM2-Sα2 within SOAR1 confers poor channel gating properties even though the chimera still avidly associates with Orai1 by virtue of its STIM1-Sα1. The single amino acid difference between STIM1-Sα2 (F394) and STIM2-Sα2 (L485) reveals the pivotal role of this residue in the Orai-activation site of STIM proteins. The F394L mutation in STIM1 substantially reduces Orai1 channel activation ( Fig. 6 ); conversely, the L485F mutation in STIM2 enhances its constitutive activation of Orai1 ( Supplementary Fig. 5 ). The relatively conservative STIM1-F394L mutation affects channel gating ( Fig. 6 ) consistent with STIM2 behaving as a partial agonist of Orai1 ( Fig. 9c,d ). The more severe STIM1-F394A substitution affects both Orai1 activation and binding, operating as a still weaker channel agonist ( Fig. 9e ). Significantly, the STIM1-F394H mutation is unable to activate or bind to Orai1 and is a complete non-agonist of Orai1 ( Fig. 9f ). That such a modest amino-acid substitution (F394H) would exact such profoundly altered function is remarkable. Likely, F394 undergoes a strategically important hydrophobic interaction with Orai1 that is prevented by the introduction of charge within the dimensionally similar histidine ring. Surprisingly, this single substitution also overrides the strong Orai1 interaction mediated by the Sα1 helix. This suggests that the apical regions of both Sα1 and Sα2 may function as a single tight Orai-interacting unit, agreeing with the recent suggestion by McNally et al. [22] that the close proximity of the M1 and M4 cytoplasmic extensions in Orai1 (ref. 16 ) creates a single binding pocket for SOAR. We suggest exposed hydrophobic residues on the Orai1 M1-extension may constitute part of this binding site ( Supplementary Fig. 6 ). Thus, in addition to defining a crucial Orai-interacting site, the results provide a new molecular understanding of the physiological distinctions between STIM1 and STIM2. The functionally pivotal Sα2 phenylalanine is replaced in STIM2 by a leucine reducing its gating efficacy. In addition, the closely associated Sα1 region has lowered binding efficacy in STIM2. However, since STIM2 has subtly lower affinity for Ca 2+ than STIM1 (ref. 29 ) and is on the ‘cusp’ of activation at resting ER Ca 2+ levels [29] , [35] , there will be more STIM2 than STIM1 in junctions under resting or partially ER-depleted conditions. Thus, under this condition, activated STIM2 in ER–PM junctions would out-compete STIM1. In earlier studies, we showed that STIM2 over expression suppresses endogenous SOCE [35] , [36] , a result that is explained by the poor efficacy of STIM2 on the Orai1 channel. The combination of increased sensitivity to Ca 2+ store-depletion and decreased Orai channel efficacy likely contributes to the different roles of STIM1 and STIM2 in receptor-induced Ca 2+ signal generation [45] , [46] . Moreover, the lower target channel efficacy of STIM2 is likely important in preventing uncontrolled Ca 2+ entry due to the near-constitutive activation of STIM2. Certainly, the competitive interaction between STIM1 and STIM2 may have special importance in those tissues with prominent STIM2 expression, including neural, cardiac, smooth muscle, pancreatic and dendritic cells [1] , [47] , [48] . DNA Constructs STIMct C-terminally YFP-labelled constructs were inserted within the pIRESneo3 plasmid (Clontech). SOAR and SOAR chimera constructs were inserted within the pEYFP-c1 plasmid (Clontech) between XhoI/EcoRI sites to create N-terminally-labelled SOAR derivatives. STIM2ct-3EA-YFP was derived from STIM2ct-YFP [41] utilizing the Quikchange II site directed mutagenesis kit (Agilent Technologies). STIM1ct-4EA-YFP was mutated from the previously described STIM1ct-YFP construct [41] . STIM2ct-ΔV-3EA-YFP was generated by deletion of the C-terminal 238 amino acids (596–833 on STIM2) on STIM2ct-3EA-YFP by PCR. STIM1ct-ΔV-4EA-YFP was generated by deletion of the C-terminal 180 amino acids (506–685 on STIM1) on STIM1ct-4EA-YFP. Constructs not generated on site were made by (Mutagenex, NJ). Cell culture and transfection Stable HEK293 expressing Orai1-CFP were derived and maintained in Dulbecco's modified Eagle's medium (Mediatech) supplemented with 10% fetal bovine serum, penicillin and streptomycin (Gemini Bioproducts, CA) (37 °C; 5% CO2) in G418 (100 μg ml −1 ) [36] , [41] . All plasmid transfections were undertaken by electroporation using the Bio-Rad Gene Pulser Xcell system in OPTI-MEM medium [41] . DNA constructs were introduced by electroporation at 180 V, 25 ms in 4 mm cuvettes (Molecular BioProducts). Transfected cells were cultured on coverslips (25 mm) in OPTI-MEM with 5% FBS and measurements undertaken 14–48 h after transfection [39] . Cytosolic Ca 2+ measurements Intracellular Ca 2+ levels were measured by ratiometric imaging using fura-2. Loading of fura-2 and imaging of fura-2 fluorescence utilized loading and fluorescence solutions comprising: 107 mM NaCl, 7.2 mM KCl, 1.2 mM MgCl 2 , 11.5 mM glucose, 20 mM Hepes-NaOH, pH 7.2 (ref. 40 ). During dye-loading, cells were treated with 2 μM fura-2/AM for 30 min at room temperature, then transferred to fura-2-free solution for a further 30 min. Ratio fluorescence imaging was measured utilizing the Leica DMI 6000B fluorescence microscope controlled by Slidebook 5.0 software (Intelligent Imaging Innovations; Denver, CO). Consecutive excitation at 340 nm ( F 340 ) and 380 nm light ( F 380 ) was undertaken every 2 s; emission fluorescence was collected at 505 nm. Intracellular Ca 2+ levels are shown as F 340 / F 380 ratios obtained from groups of 5–35 single cells on coverslips. All Ca 2+ imaging experiments were undertaken at room temperature and representative traces of at least three independent repeats are shown as mean±s.e.m. Förster resonance energy transfer measurements To determine FRET signals between stably expressed Orai1-CFP and transiently expressed YFP-tagged STIM fragments, we used the Leica DMI 6000B fluorescence microscope equipped with CFP (438 Ex /483 Em ), YFP (500 Ex /542 Em ), FRET raw (438 Ex /542 Em ) filters. Images captured with the CFP, YFP and FRET filters ( F CFP , F YFP and F raw , respectively) were collected every 20 s at room temperature using a × 40 oil objective (N.A.1.35; Leica) and processed using Slidebook 5.0 software (Intelligent Imaging Innovations). Three-channel corrected FRET was calculated using the following formula: FRET c = F raw − F d / D d * F CFP − F a / D a * F YFP where FRET c represents the corrected energy transfer, F d / D d represents measured bleed-through of CFP through the YFP filter (0.447), and F a / D a is measured bleed-through of YFP through the CFP filter (0.049). Although the CFP signal was constant in Orai1-CFP stable cells, there was some variation in transiently expressed YFP levels. To compensate for these variations in YFP expression, the above FRET c values were normalized against acceptor fluorescence ( F YFP ) to generate ‘N-FRET’ signals. Thus, N-FRET=FRET c / F YFP . In some figures, the relative changes in N-FRET were compared with resting N-FRET (N-FRET rest ) levels. This is denoted as ΔN-FRET/N-FRET rest , in which ΔN-FRET=N-FRET—N-FRET rest . Average FRET measurements shown are typical of at least three independent analyses ±s.e.m. Enhanced Fluorescence Image Analysis Enhanced images of the cellular distribution of fluorescently-tagged STIM and Orai constructs were obtained from stacks of 10–20 3-D Z-axis image-planes collected at 1 μm steps. The constrained iterative deconvolution function of the Slidebook 5.0 software was used to analyse image stacks and derive enhanced deconvolved images with minimized fluorescence contamination from out-of focus planes. STIM and Orai images shown were typical of at least three independent experiments. Analysis of STIM and Orai Fluorescence Intensity in Puncta Levels of STIM1 and Orai1 within punctal regions were quantified by comparing YFP or CFP fluorescence in punctal regions, and in corresponding adjacent control regions. Average wild-type or mutant STIM1-YFP fluorescence within puncta (YFP puncta ) and adjacent control areas (YFP control ) were exported using the ‘ratio/timelapse-data’ function in Slidebook. The ratio of YFP puncta /YFP control was used to define the relative enrichment of STIM1 in puncta after ionomycin. Levels of Orai1-CFP were measured in the same superimposed punctal and adjacent control regions selected from the STIM-YFP images, to give CFP puncta /CFP control . The relative changes (Δ) are shown compared with resting levels before ionomycin application. Analyses shown are from six cells taken from three independent experiments, with 20–30 punctal and control regions selected from each cell. Electrophysiological measurements Conventional whole-cell recordings in HEK-Orai1 cells transiently expressing STIM1 or its mutants were performed [39] . After establishing whole-cell configuration, a 50 ms voltage step (−100 mV) from a holding potential of 0 mV, followed by a voltage ramp spanning from −100 to +100 mV in 50 ms was delivered every 2 s. The intracellular solution contained: 135 mM Cs aspartate, 8 mM MgCl 2 , 8 mM BAPTA, and 10 mM Cs-HEPES (pH 7.2). The extracellular solutions contained: 130 mM NaCl, 4.5 mM KCl, 20 mM CaCl 2 , 10 mM TEA-Cl, 10 mM D -glucose, and 5 mM Na-HEPES (pH 7.4). A 10 mV junction potential compensation was applied to correct the liquid junction potential between pipette solutions relative to extracellular solution. All whole-cell currents were filtered at 3.3 kHz and sampled at 10 kHz. Western analyses Cells were lysed in cell lysis buffer containing 50 mM Tris–HCl, pH 8.0, 150 mM NaCl, 1% IGEPAL CA‐630, and 100 μM phenylmethylsulfonyl fluoride and 5% protease inhibitor cocktail (Sigma-Aldrich). Lysis took place on ice for 30 min, followed by centrifugation at 14,000 g , 4 °C for 10 min. Supernatants were quantified using Bio-Rad DC protein assay kits. Protein extracts (20 μg per lane of each) were resolved on 8% SDS-polyacrylamide gels and electroblotted onto Bio-Rad Immun-Blot PVDF membranes. After transfer, the PVDF membranes were blocked in Tris-buffered saline-Tween 20 (TBST; containing 10 mM Tris–HCl, pH 8.0, 150 mM NaCl, 0.05% Tween 20) containing 5% BSA (Sigma-Aldrich) for 1 h at room temperature, then incubated with Rabbit GFP primary antibody (dilution 1:1000) overnight at 4 °C. Membranes were washed two times (7 min) in TBST and incubated with secondary antibody (Anti-Rabbit immunoglobulin G (H+L) from KPL, Inc.) and Precision Protein StrepTactin-horseradish perioxidase conjugate (Bio-Rad) for 30 min. Subsequently, membranes were washed three times (5 min) in TBST. Peroxidase activity was examined with SuperSignal West Pico Chemiluminescent Substrate (Thermo Scientific) using the manufacturer’s protocols; the resulting fluorescence was collected using an Alpha Inotech MultiImage II system. Immunoprecipitation Cells were treated as indicated in the legend and lysed in chilled lysis buffer containing 150 mM NaCl, 10 mM Tris–HCl (pH 7.4), 1% Igepal Ca-360, and one tablet of complete protease inhibitors (Santa Cruz, sc-29131) per 25 ml. For 2-APB treatment, lysis buffer was supplemented with 50 μM 2-APB. Cell lysates were centrifuged (14,000 g , 10 min at 4 °C). After quantification with Bio-Rad DC protein assay kits, 500 μg cell lysate samples (2 μg μl −1 ) were incubated with protein G agarose (Invitrogen, 15920-010) for 10 min at 4 °C. Input samples were prepared from preincubated cell lysates (whole-cell lysate), the remaining lysates were immunoprecipitated with sheep anti-STIM1 antibody (2 μl per sample) by rotation for 2 h at 4 °C, followed by an additional 1 hr incubation with protein G agarose. Sheep anti-STIM1 antibody was purified from a polyclonal anti-STIM1 serum [39] . The precipitates were washed three times with lysis buffer and eluted in gel-loading buffer by heating at 100 °C for 10 min, and resolved in 4–12% NuPAGE Bis-Tris gels. Proteins of interest were immunoblotted using anti-GFP (1 μg ml −1 , Santa Cruz, sc-9996), anti-Orai1 (1 μg ml −1 , Sigma, O8264), or anti-GAPDH (1:1000, Proteintech, 60004-1-Ig) antibody. To minimize immunoglobulin G contamination from primary antibodies used in immunoprecipitation, clean-blot IP detection reagent (horseradish perioxidase; Thermo Scientific, 21232) was applied. Peroxidase activity was visualized using the ECL kit (Thermo Scientific, SuperSignal West Femto Chemiluminescent Substrate) with the FluorChem HD2 imaging system from Alpha Innotech. Original membrane scans are provided in Supplementary Fig. 3 . Homology modelling The SOAR2 domain of the STIM2 protein was modelled as a dimer using Biological Assembly Modeler (BAM, version 2.0) which allows simultaneous modelling of both chains based on a single template ( http://dunbrack.fccc.edu/BAM ; Maxim V. Shapovalov, Qiang Wang, Qifang Xu, and Roland L. Dunbrack, Jr.) (PDB code 3TEQ). Modelling also utilized MolIDE software [49] . Side-chain rotamers for the dimer were optimized with a backbone dependent library and the SCWRL 4 software [50] , [51] . Superpositioning of the SOAR2 model with the SOAR1 structure was undertaken using the Chimera software [52] that was also used to prepare figures. Statistical analyses Analysis of statistical significance was performed using unpaired Student’s t -test with GraphPad Prism 5 software. Results are expressed as means±s.e.m., ** P <0.01; *** P <0.001. How to cite this article : Wang, X. et al. Distinct Orai-coupling domains in STIM1 and STIM2 define the Orai-activating site. Nat. Commun. 5:3183 doi:10.1038/ncomms4183 (2014).